Doping strain induced bi-Ti3+pairs for efficient N2activation and electrocatalytic fixation The electrochemical N 2 fixation to produce ammonia is attractive but significantly challenging with low yield and poor selectivity. Herein, we first used density function theory calculations to reveal adjacent bi-Ti 3+ pairs formed on anatase TiO 2 as the most active electrocatalytic centers for efficient N 2 lying-down chemisorption and activation. Then, by doping of anatase TiO 2 with Zr 4+ that has similar d -electron configuration and oxide structure but relatively larger ionic size, the adjacent bi-Ti 3+ sites were induced and enriched via a strained effect, which in turn enhanced the formation of oxygen vacancies. The Zr 4+ -doped anatase TiO 2 exhibited excellent electrocatalytic N 2 fixation performances, with an ammonia production rate (8.90 µg·h −1 ·cm −2 ) and a Faradaic efficiency of 17.3% at −0.45 V versus reversible hydrogen electrode under ambient aqueous conditions. Moreover, our work suggests a viewpoint to understand and apply the same-valance dopants in heterogeneous catalysis, which is generally useful but still poorly understood. The production of ammonia (NH 3 ) by the well-known Haber‒Bosch process from N 2 and H 2 has marked over a century of success for providing > 80% nitrogen source for fertilizer and an alternative energy carrier with large energy density [1] . Despite the natural abundance of N 2 , the high bond energy of the N≡N triple bond (941 kJ mol −1 ) prevents it as a reactive form and thus demands a significant amount of the global energy cost annually [2] . In addition, the use of fossil fuels to produce H 2 reactant also leads to a significant level of CO 2 release [3] . The electrochemical N 2 fixation (also known as N 2 reduction reaction, N 2 RR) can be processed in ambient conditions and use inexpensive aqueous electrolytes as the proton source, and thus is regarded as a promising alternative approach [4] . The direct electron transfer from electrode surface to N ≡ N requires overcoming substantially high energy barriers [5] , so the key to achieve efficient N 2 fixation is to develop active catalytic centers that can efficiently reduce the large activation barrier of N ≡ N and promote its dissociation. As an overwhelming level of water molecules exists than solvated N 2 , the other key to achieve this goal is to enrich the electrocatalytic centers that can favorably proceed with the N 2 RR over the hydrogen evolution reaction (HER). Theoretical calculations have suggested that metal sites with low chemical valence are potential to enhance the electron-donating ability to the π* antibonding orbitals of N 2 molecule [6] , which weakens the N≡N bond and drives the eventual cleavage of N 2 . Some noble metal-based catalysts such as Ru [7] and Au [8] with stepped surfaces can strongly bind to N 2 and the intermediates, and thus can lower the overpotential and increase the rate of the N 2 RR in an aqueous electrolyte. Earth-abundant compounds [4] , [9] , including metal oxides, nitrides and carbides, have also been investigated as electrocatalysts [10] , with tailorable activities by specific facets [11] , defects [12] , vacancies [13] , or hybrid material interfaces [14] . Nonetheless, to date, the electrocatalytic N 2 fixation is still limited by its low yields and slow kinetics [15] . The critical understanding and rational tuning the active centers of N 2 RR electrocatalysts remain as a highly challenging but imperative issue. Previously, the roles of oxygen vacancies (Vo’s) in transition metal oxides have been extensively discussed [16] , [17] , [18] , and the low-valance dopants have also been suggested to facilitate the formation of Vo’s [19] , but the knowledge of their contributions to the N 2 RR is still limited. For example, Li et al. reported that TiO 2 with Vo’s can chemisorb and activate N 2 molecules [16] , and the formation of each Vo’s is, in turn, related to the formation of a pair of Ti 3+ . Hirakawa et al. [17] suggested that two Ti 3+ ions in adjacent positions, which are inherently created on the surface defects of rutile TiO 2 (110) surfaces, behave as active sites for photocatalytic conversion of N 2 to ammonia with water. However, more-recent calculations provide different results and indicate that such rutile TiO 2 (110) surfaces are unlikely to be the relevant surface for the N 2 RR [20] . To date, all the theoretical and experimental studies have not been able to reconcile the discrepancies in which types of TiO 2 are the best for the N 2 RR, or what is the bonding nature of the active centers. Herein, by means of density function theory (DFT) calculations, we first reveal that two adjacent Ti 3+ sites (designated as a bi-Ti 3+ pair) on anatase TiO 2 (101) can chemically adsorb and activate N 2 molecules in a lying-down manner, whereas single or isolated Ti 3+ sites cannot. On the other hand, similar bi-Ti 3+ pair on rutile (110) surface cannot adsorb and activate N 2 , unless the strong repulsion between one of its nearest lattice oxygens at the bridge sites and the negatively charged N 2 upon activation can be eliminated. Thus, the formation of two adjacent Ti 3+ sites on anatase (101) should be the most-effective electrocatalytic centers for N 2 fixation. Accordingly, we develop an experimental strategy for inducing such adjacent bi-Ti 3+ sites on anatase (101) surfaces as N 2 RR active centers, using a dopant-induced Vo formation strategy. Zr 4+ is selected to dope in the TiO 2 framework, owing to its similar d -electron configuration and oxide structure, as well as its suitable size. As shown in Fig. 1 , doping of Zr 4+ , which has a relatively larger radius of 72 pm (compared with 52 pm of Ti 4+ ) [21] into anatase TiO 2 , can still retain its anatase crystal structure but also exert a tension on the TiO 2 framework, which can enhance the formation of Vo. As the oxidation number of Zr 4+ is fixed, the newly formed Vo must be associated with the formation of two adjacent Ti 3+ sites, which are beneficial to enrich active centers and enhance the N 2 RR over the HER. In contrast, Ce 4+ with a much larger ion radius (106 pm) cannot be incorporated into the TiO 2 framework without breaking the original crystal structure, whereas Ce 3+ can also be associated with the newly formed Vo’s, thus not contributing to the formation of the bi-Ti 3+ pairs as active centers. Electrochemical measurements demonstrate that the Zr 4+ -doped anatase TiO 2 exhibit significant enhanced N 2 RR performances, including an ammonia formation rate of 8.90 ± 0.17 µg h −1 cm −2 catalyst and a corresponding Faradaic efficiency (FE NH3 ) of 17.3%, significantly surpassing those of undoped TiO 2 or Ce 4+ -doped TiO 2 , whose efficiencies were limited by their lower Ti 3+ densities. Fig. 1 Schematic illustration of N 2 fixation and activation. a The formation of an oxygen vacancy (Vo) and adjacent bi-Ti 3+ sites owing to the Zr-doping in anatase TiO 2 . b Comparison of the ionic radius of Ti 4+ , Ti 3+ , and Zr 4+ Full size image Theoretical calculations In order to tune Ti 3+ -based electrocatalysts for the N 2 RR, DFT calculations were first carried out to rationally screen different types of Ti 3+ for a better understanding of bonding structures of these active centers. The calculations for screening an ideal N 2 RR electrocatalyst are often based on the following criteria: [22] , [23] , [24] first, strong chemisorption of N 2 molecules; second, effective stabilization of N 2 H*; and third, destabilization of NH 2 *. In the present study, we also investigated the capability of forming Vo’s efficiently, as the fourth criterion. According to the four criteria above, several types of Ti 3+ sites were screened for the N 2 RR, including adjacent bi-Ti 3+ pairs on anatase (101) surfaces (designated as A(101)-Vo), rutile (110) surfaces with 1 or 2Vo’s (designated as R(110)-Vo, R(110)-2Vo, respectively), as well as single Ti 3+ with four coordination sites on anatase (101) surfaces (Fig. 2 ). As shown below, the number of the associated Vo’s is critical to discriminate against the active and non-active bi-Ti 3+ sites. We utilized density functional theory (DFT) and the computational hydrogen electrode (CHE) approach [25] that have been proven useful in understanding various electrocatalytic reactions [20] , [22] , [26] , [27] , [28] . More details about how to determine the active sites and the atomic configurations of different Ti 3+ sites are further illustrated in the Methods section, and the corresponding results are presented in Fig. 3 , Supplementary Fig. 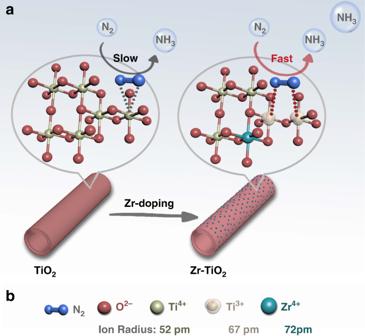Fig. 1 Schematic illustration of N2fixation and activation.aThe formation of an oxygen vacancy (Vo) and adjacent bi-Ti3+sites owing to the Zr-doping in anatase TiO2.bComparison of the ionic radius of Ti4+, Ti3+, and Zr4+ 1 and Supplementary Table 1 . Fig. 2 DFT calculations of four types of Ti 3+ sites. a The adjacent bi-Ti 3+ on anatase (101) surfaces with one oxygen vacancy (i.e., A(101)-Vo); b the single Ti 3+ with four coordination on anatase (101) surfaces with one oxygen vacancy; c the adjacent bi-Ti 3+ on rutile (110) surfaces with one oxygen vacancy (i.e., R(110)-Vo); d the adjacent bi-Ti 3+ on rutile (110) surfaces with a pair of oxygen vacancies together, (i.e., R(110)-2Vo’s). The light-blue spheres stand for the lattice oxygens at the bridge sites where the surface oxygen vacancies are formed most easily. The red spheres stand for the other lattice oxygens on the surfaces and the gray spheres stand for the titanium cations. All four types of the active site models are highlighted by using the green circles. As compared c and d , the bridge lattice oxygen (circled in blue) can exert a large repulsion with the chemisorbed N 2 if it adopts a lying-down mode Full size image Fig. 3 DFT predicted activity for different types of Ti 3+ site. a adjacent bi-Ti 3+ on anatase (101) surfaces with oxygen vacancy, b single Ti 3+ on anatase (101) surfaces with oxygen vacancy. The light-blue spheres stand for the lattice oxygens at the bridge sites where the surface oxygen vacancies are formed most easily. The red spheres stand for the other lattice oxygens on the surfaces and the gray spheres stand for the titanium cations. Δ G refers to the free energy, and Δ E refers to the electronic energy. The Vo formation energy, Δ E (Vo), was calculated in related to the 1/2 O 2 formation as described in the Methods section Full size image The adsorption of N 2 molecule is the first step to initialize the N 2 RR [22] , [23] , [29] . Both the adsorption free energy (Δ G ) and the adsorption electronic energy (Δ E ) are presented in Fig. 3 and Supplementary Fig. 1 . As free N 2 has a very stable triple bond, whereas the charge transfer and bond elongation are associated with high energy cost, these quantities are used as a strong evidence to show whether or not N 2 is chemisorbed and activated. The A(101)-Vo (i.e., Vo on anatase (101) planes) presents adjacent bi-Ti 3+ pairs, which can effectively induce the chemisorption of N 2 in a lying-down manner and subsequent activation (Fig. 3a ). This is illustrated by the fact that N 2 molecule is 0.56 |e| charged (Bader charge [30] ), which makes the N−N bond length elongated from 1.12 Å in an original N 2 molecule to 1.18 Å in the chemisorbed state. Similar chemisorption of N 2 was also reported on the Vo’s of anatase (010) [17] . On the contrary, the adjacent bi-Ti 3+ pairs on R(110)-Vo (Supplementary Fig. 1a ) and single Ti 3+ sites on the A(101)-Vo (Fig. 3b ) can only adsorb N 2 in a standing-up manner, with much less charge transfer and negligible N−N bond length elongation. Furthermore, by comparing the geometry structures between the adsorbed N 2 on R(110)-Vo and that on A(101)-Vo, it can be seen that there exists a large repulsion in the former between the adsorbed N 2 and one of the adjacent lattice oxygens at the bridge site, owing to a close distance between negatively charged N and the lattice O 2‒ (Fig. 2 and Supplementary Fig. 1a ). Thus, it is only when such lattice O 2‒ is removed and an adjacent bi-Ti 3+ pair on R(110)-2Vo is formed, the efficient activation of N 2 can occur as shown by a significant amount of negative charge on N 2 and an elongated N−N bond length (Supplementary Fig. 1b ). Based on the aforementioned Criterion 2 , the first hydrogenation step was further investigated. The results show that the initial N 2 adsorption has a large impact on the subsequent hydrogenation. As illustrated in Fig. 3a and Supplementary Fig. 1b , the calculated reaction free energies (Δ G ) for the first hydrogenation step on A(101)-Vo and R(110)-2Vo are 0.24 and 0.25 eV, respectively, much lower than those on the single Ti 3+ sites (0.50 eV, Fig. 3b ) and the adjacent bi-Ti 3+ sites on R(110)-Vo (0.75 eV, Supplementary Fig. 1a ), whereas N 2 is also inactivated in the latter two cases. Our calculation results agree with the previous hypothesis [20] , and show that R(110)-Vo is unlikely to be the relevant surface for the N 2 RR. Here, we can now rule out the two configurations of single Ti 3+ sites and the adjacent bi-Ti 3+ sites on R(110)-Vo, which cannot activate N 2 and are unfavorable for the first hydrogenation step. By examining the Criterion 3 , we found that the reaction free energies for the hydrogenation of NH 2 * on A(101)-Vo (Fig. 3a ) and R(110)-2Vo (Supplementary Fig. 1b ) are 0.18 and 0.23 eV, respectively. These numbers can be favorably compared with those for the first hydrogenation step. Hence, following the first three criteria, both the adjacent bi-Ti 3+ pair sites on A(101)-Vo and R(110)-2Vo are active for the N 2 RR. However, as shown in Supplementary Fig. 1a and b, the formation of two adjacent Vo’s on rutile (110) surfaces is 0.36 eV higher than the formation of two separated Vo’s (see more discussion in the Methods section). This downplays the role of the adjacent bi-Ti 3+ sites on R(110)-2Vo. Hence, the anatase (101) surface is the more suitable support for the development and enrichment of the active bi-Ti 3+ pair sites. The feasibility of the N 2 RR on the adjacent bi-Ti 3+ on A(101)-Vo is also confirmed by the whole free energy pathway calculated at 0 and −0.24 V as presented in Supplementary Fig. 2 . Low-valance dopants have often been utilized to facilitate the formation of Vo’s [19] . However, their incorporation into TiO 2 does not guarantee the formation and enrichment of the active bi-Ti 3+ sites. On the other hand, the same-valance dopants are generally useful in heterogeneous catalysis [19] , whereas their roles are less understood. Assuming that the same-valance dopants could introduce strain into the original lattice, we examined how lattice expansion and contraction would change the formation energy of Vo’s. As shown in Supplementary Fig. 3 , both the tensile strain and the compressive strain can lower the formation energy of Vo’s in the anatase lattice (see the Methods for more computational details). Considering Ti 4+ is the smallest cation for the oxidation state of M 4+ (e.g., 72 pm of Zr 4+ , or 106 pm of Ce 4+ , as compared with 52 pm of Ti 4+ ) [21] , introducing the tensile strain is practically feasible. Note that Zr 4+ has a similar d -electron configuration and oxide structure, it is thus an ideal replacement of Ti 4+ . Furthermore, as the oxidation number of Zr 4+ is fixed, the newly formed Vo’s are expected to be associated with the formation of two adjacent Ti 3+ , which are beneficial to the enrichment of the active sites. In contrast, Ce 4+ has a much larger ion radius (106 pm), presumably lowering the formation energy of Vo’s to a larger extent. Nevertheless, it is more likely to break the original crystal structure of TiO 2 upon Ce 4+ doping. Furthermore, Ce 4+ can be reduced to Ce 3+ during the formation of Vo’s [21] , and thus does not contribute to the formation of the bi-Ti 3+ active centers upon doping. Synthesis and structural characterizations TiO 2 anatase nanotubes were first synthesized by a hydrothermal method, followed by incubation of Zr 4+ or Ce 4+ dopants with subsequent annealing (see Methods section). The crystal structures of different samples were investigated by X-ray diffraction (XRD, Fig. 4a ). For the undoped and Zr 4+ -doped TiO 2 (designated as Zr-TiO 2 ) nanotubes, all the diffraction peaks correspond to an anatase phase (JCPDS# 21‒1272). The TiO 2 peak intensity decreases with the Zr 4+ doping, suggesting the slight decrease of TiO 2 crystallinity, but no peaks associated with ZrO 2 are observed. Close examination of the spectra shows that with the increasing Zr 4+ content, the XRD peaks gradually shift toward lower diffraction angles (Fig. 4b ), indicating the increase of TiO 2 lattice constants upon Zr 4+ doping. The corresponding interplanar spacing values of the (101) planes change from 0.351 nm for undoped TiO 2 to 0.359 nm for Zr-TiO 2 . 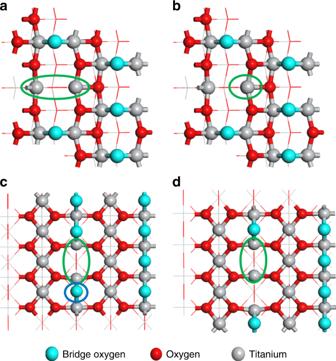Fig. 2 DFT calculations of four types of Ti3+sites.aThe adjacent bi-Ti3+on anatase (101) surfaces with one oxygen vacancy (i.e., A(101)-Vo);bthe single Ti3+with four coordination on anatase (101) surfaces with one oxygen vacancy;cthe adjacent bi-Ti3+on rutile (110) surfaces with one oxygen vacancy (i.e., R(110)-Vo);dthe adjacent bi-Ti3+on rutile (110) surfaces with a pair of oxygen vacancies together, (i.e., R(110)-2Vo’s). The light-blue spheres stand for the lattice oxygens at the bridge sites where the surface oxygen vacancies are formed most easily. The red spheres stand for the other lattice oxygens on the surfaces and the gray spheres stand for the titanium cations. All four types of the active site models are highlighted by using the green circles. As comparedcandd, the bridge lattice oxygen (circled in blue) can exert a large repulsion with the chemisorbed N2if it adopts a lying-down mode 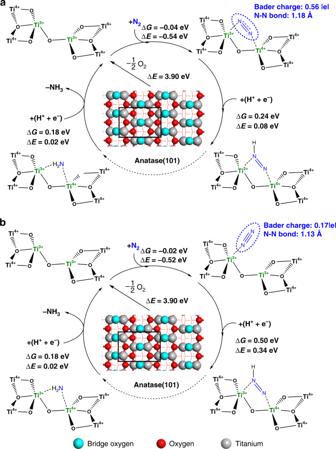Fig. 3 DFT predicted activity for different types of Ti3+site.aadjacent bi-Ti3+on anatase (101) surfaces with oxygen vacancy,bsingle Ti3+on anatase (101) surfaces with oxygen vacancy. The light-blue spheres stand for the lattice oxygens at the bridge sites where the surface oxygen vacancies are formed most easily. The red spheres stand for the other lattice oxygens on the surfaces and the gray spheres stand for the titanium cations. ΔGrefers to the free energy, and ΔErefers to the electronic energy. The Vo formation energy, ΔE(Vo), was calculated in related to the 1/2 O2formation as described in the Methods section This observation of anatase TiO 2 lattice expansion upon the Zr 4+ doping is supported by the DFT calculations (Supplementary Table 2 and Supplementary Table 3 ). In contrast, the Ce-doped TiO 2 does not exhibit characteristic peaks of TiO 2 , but presents peaks that are associated with CeO 2 (JCPDS# 43‒1002), suggesting the loss of TiO 2 anatase structure and the formation of CeO 2 crystals upon the Ce 4+ doping. As a comparison, the Zr 4+ doping on rutile TiO 2 (designated as Zr-rutile-TiO 2 ) was also conducted to illustrate the effect of different active sites. The XRD peaks (Supplementary Fig. 4 ) confirm the typical rutile phase (JCPDS# 21‒1276). Fig. 4 Structural and compositional characterizations. a X-ray diffraction (XRD) patterns of ZrO 2 , CeO 2 , undoped TiO 2 , Ce-TiO 2 , and Zr-TiO 2 . b The enlarged view of XRD pattern at 22 o −28 o range. c – e High-resolution transmission electron microscopy (HRTEM) images of c undoped TiO 2 , d Ce-TiO 2 , and e Zr-TiO 2 samples. Insets: Transmission electron microscopy (TEM) images of the corresponding nanotubes. f High-angle annular dark-field scanning transmission electron microscopy (HAADF-STEM) image with corresponding element mappings of Zr-TiO 2 , showing the distribution of Ti (green), O (blue), and Zr (red). (Source data are provided as a Source Data file.) Full size image High-resolution transmission electron microscopy images show that the undoped (pristine) TiO 2 anatase nanotubes have a tubular structure, with the outer and inner diameters of 7–9 and ~ 4 nm, respectively (Fig. 4c ). The resolved lattice fringes are measured as 0.351 nm, consistent with the interplanar distance of (101) planes of anatase TiO 2 . After doping with 5% Ce 4+ (i.e., Ce-TiO 2 , Fig. 4d ), small CeO 2 nanoparticles are observed on the exteriors of original TiO 2 nanotubes, suggesting an inhomogeneous behavior of phase separation. In contrast, for TiO 2 nanotubes doped with 5% Zr 4+ (i.e., Zr-TiO 2 , Fig. 4e ), no nanoparticles are observed outside the nanotubes. The resolved lattice fringes of 0.359 nm are similar but slightly larger than those of (101) planes of anatase TiO 2 , also in good accord with the XRD results. The energy-dispersive X-ray spectroscopy (EDS) and mapping confirm the existence and uniform distribution of Ti, O, and Zr elements in the nanotubes (Fig. 4f and Supplementary Fig. 5 ). High-angle annular dark-field scanning transmission electron microscopy (HAADF-STEM) was then used to characterize the dopant distribution in different types of TiO 2 nanotubes. Compared with the undoped TiO 2 nanotubes (Fig. 5a ), individual Zr 4+ ions are observed to occupy the original positions of Ti 4+ , exhibiting a distribution of single atoms (highlighted by red circles in Fig. 5b ). The electron energy loss spectroscopy (EELS) analysis of Ti-edge was conducted to probe the phase and chemical states of titanium for the undoped, Zr- and Ce-doped TiO 2 nanotubes, respectively (Fig. 5c ). The undoped TiO 2 nanotubes present Ti 4+ features with two peaks at 458.4 (Ti-L 3 ) and 463.7 eV (Ti-L 2 ), respectively. For Zr-TiO 2 , the centers of these two peaks shift to lower energy near 457.5 and 462.7 eV, respectively, indicating that the cation incorporation elevates the content of the unoccupied Ti 3 d state as well as the distorted Ti 3+ coordination [31] . Furthermore, a shift of 0.6 eV to lower energy is observed for the Ti-L 3 edge in the EELS spectra of Ce-TiO 2 , associating with the existence of a distorted structure in Ce-TiO 2 samples [31] . Based on the intensity of L 2 and L 3 from the Zr-TiO 2 sample (Supplementary Fig. 6a ), the ratio of Ti 3+ /∑Ti (∑Ti = Ti 3+ + Ti 4+ ) is estimated to be 29.1% [32] . Similarly, the Ti 3+ /∑Ti values of undoped TiO 2 and Ce-TiO 2 are calculated as 8.5% and 21.0%, respectively (Supplementary Fig. 6b, c ). Fig. 5 Structural and compositional characterizations. High-angle annular dark-field scanning transmission electron microscopy (HAADF-STEM) of a undoped TiO 2 and b Zr-TiO 2 samples. Single Zr 4+ ions were highlighted by red circles. c Electron energy loss spectroscopy (EELS) profiles of the Ti-L 2, 3 edge recorded across the undoped TiO 2 , Ce-TiO 2 , and Zr-TiO 2 samples. d Ti 2p X-ray photoelectron spectroscopy (XPS) spectra of the Zr-TiO 2 , Ce-TiO 2 , and undoped TiO 2 , samples. (Source data are provided as a Source Data file.) Full size image X-ray photoelectron spectroscopy (XPS) was further conducted to study the oxidation states of metal ions on the catalyst surfaces. For the undoped TiO 2 nanotubes (Fig. 5d , bottom panel), two main peaks centered at 458.9 and 464.6 eV are observed, corresponding to the Ti 2p 3/2 and Ti 2p 1/2 peaks, respectively. These two peaks can be further deconvoluted into four sub-peaks, assigned to Ti 3+ 2p 3/2 (457.4 eV), Ti 4+ 2p 3/2 (458.9 eV), Ti 3+ 2p 1/2 (463.1 eV), and Ti 4+ 2p 1/2 (464.6 eV), respectively, confirming the coexistence of Ti 3+ and Ti 4+ species [33] . The ratio between Ti 3+ and ∑Ti for undoped TiO 2 is calculated as 10%. The incorporation of Zr 4+ into TiO 2 frameworks leads to a clear shift to lower binding energy direction and widening both peaks (Fig. 5d , top panel), suggesting the increase of the Ti 3+ content. The Ti 3+ /∑Ti ratio is calculated as 31% for Zr-TiO 2 nanotubes, in which the increase of Ti 3+ percentage is a clear indication of oxygen vacancy increase [34] . In comparison, the Ti 3+ /∑Ti ratio for Ce-TiO 2 nanotubes is measured as 21% (Fig. 5d , middle panel), which can be attributed to the loss of TiO 2 anatase structure, in good accord with XRD results. Accordingly, the analyses of both the Zr 3 d peaks (Supplementary Fig. 7a ) and Ce 3 d peaks (Supplementary Fig. 7b ) confirm the existence of Zr 4+ and Ce 4+ /Ce 3+ in the Zr-TiO 2 and Ce-TiO 2 nanotubes, respectively. The defects of unpaired electrons in materials were also probed by electron paramagnetic resonance spectra. Among the three samples (Supplementary Fig. 8 ), the Zr-TiO 2 sample presents the largest signal at g = 2.003, further confirming its largest concentration of Ti 3+ ions [35] . To further verify their electronic structures, these samples were characterized by X-ray Absorption Near-edge Fine Structure (XANES) spectroscopy. The XANES spectra of Ti K -edge in Zr- or Ce-doped TiO 2 samples are similar to that in undoped TiO 2 (Supplementary Fig. 9 ), confirming similar local structure modification of Ti cations [36] . The main Ti pre-edge peak at 4970.9 eV (indicated by the black arrow) in the three samples (Fig. 6a ) is ascribed to the weak symmetry of the surrounding Ti cations in these catalysts [37] . The slight increase of the pre-edge intensity in both Zr-TiO 2 and Ce-TiO 2 indicates the existence of more distorted structures and defective Ti environment [38] . The main peak of Ti K -edge at 4987.6 eV in Zr- or Ce-doped TiO 2 samples (Fig. 6b , indicated by the black arrow) is lower than that in pure TiO 2 (4987.3 eV), indicating that the Ti species are partially reduced after doping. The bond length information of different samples was further investigated by the Fourier transformed (FT) k 3 -weighted of Ti K -edge Extended X-ray Absorption Fine Structure (EXAFS) spectra (Fig. 6c ). The undoped TiO 2 nanotubes show two peaks at 1.39 and 2.41 Å, corresponding to the Ti–O and Ti–Ti bonds, respectively [39] . Interestingly, the doping of relatively larger Zr 4+ in the TiO 2 framework results in a contracted Ti–O bond length (1.34 Å) with a larger distribution, suggesting that Zr 4+ cations are interstitially incorporated in TiO 2 lattice and result in abundant surface defect sites [40] . This observation is consistent with a previous report that the contracted Ti–O bonds associated with coordinately unsaturated Ti cations acted as Lewis acid sites [41] . Fig. 6 X-ray absorption spectroscopy characterizations. a , b Enlarged Ti K -edge X-ray absorption near-edge structure (XANES) spectra, and c Fourier transformed (FT) k 3 -weighted of Ti K -edge Extended X-ray Absorption Fine Structure (EXAFS) spectra of the undoped TiO 2 , Zr-TiO 2 , and Ce-TiO 2 samples. d Zr K -edge XANES spectra and e Fourier-transformed k 3 -weighted of EXAFS spectra of pure ZrO 2 and Zr-TiO 2 samples. (Source data are provided as a Source Data file.) Full size image The Zr K -edge spectra of Zr 4+ -doped TiO 2 nanotubes were also investigated to probe the local structure surrounding Zr cations (Fig. 6d ). The main Zr K -edge in the range of 18,020–18,040 eV is split into two peaks at 18,018.5 eV (Peak A) and 18,030.0 eV (Peak B), indicating six-coordinated Zr 4+ cations that are consistent with the coordination of Ti 4+ in anatase TiO 2 structure [42] . These features are distinctively different from those of pure tetragonal ZrO 2 with 7- or 8-coordinated Zr 4+ cations [43] . The EXAFS spectra of Zr-TiO 2 (Fig. 6e ) only present the bond length of Zr–O (1.52 Å) but not Zr–Zr (3.20 Å), in agreement with the HAADF-STEM results that the Zr 4+ cations in the TiO 2 framework exhibit a single-atomic distribution. Electrochemical N 2 fixation The nitrogen temperature-programmed desorption (N 2 -TPD) was first carried out to evaluate the capability of N 2 adsorption by these samples (Supplementary Fig. 10 ). The two broad peaks centered at 170 and 500 °C are attributed to physisorption and chemisorption of N 2 , respectively [44] . Both the undoped TiO 2 and Ce-TiO 2 show very weak chemisorption peaks. In contrast, the Zr-TiO 2 sample presents a strong N 2 chemisorption, suggesting that the incorporation of Zr 4+ in the anatase TiO 2 lattice leads to a significant increase of active sites for N 2 adsorption. The aqueous electrocatalytic N 2 reduction was then conducted in an electrochemical cell at room temperature and pressure. N 2 gas was supplied in a feed gas stream to the cathode, while 0.1 m KOH aqueous solution was used as the electrolyte (Methods section). All the voltages reported in this work were converted into values versus reversible hydrogen electrode (vs. RHE), as shown in Supplementary Fig. 11 . The linear sweep voltammetric (LSV) curves of the Zr-TiO 2 nanotubes were first measured in both N 2 -saturated and Ar-saturated electrolytes, respectively, in the same voltage range (Fig. 7a ). A clear current density increase is observed for the N 2 -saturated electrolyte, suggesting the occurrence of the N 2 RR [11] . The thermodynamic equilibrium potential of N 2 to NH 3 in 0.1 m KOH is calculated as 0.056 V vs. RHE (detailed calculation shown in the Supplementary Note 1 ), based on the free energies tabulated in literature [45] . Here, the onset potential of the overall electrochemical reactions is defined as the total current density gets over 50 μA cm ‒2 . In order to achieve this current density, the onset potentials of the undoped TiO 2 , Ce-TiO 2 , Zr-rutile-TiO 2 , and Zr-TiO 2 catalysts are ‒ 0.246, ‒ 0.178, ‒ 0.497, and ‒ 0.141 V vs. RHE, respectively (Supplementary Fig. 12 and Supplementary Fig. 13 ). For a current density of 1 mA cm ‒2 achieved, the undoped TiO 2 , the Ce-TiO 2 , Zr-rutile-TiO 2 , and Zr-TiO 2 require ‒ 0.643, ‒ 0.578, ‒ 0.715, and ‒ 0.538 V vs. RHE, respectively. This comparison suggests that the incorporation of Zr 4+ should be the main contributor of active sites for catalyzing N 2 RR. The partial current densities for ammonia production were calculated by multiplying the total current density with the FE NH3 at selected potentials (Supplementary Fig. 14 ). By defining the current density level toward NH 3 production as 25 μA cm ‒2 , the N 2 RR onset potential for the Zr-TiO 2 is calculated as ‒ 0.4 V vs. RHE, corresponding to the overpotential of 456 mV. Fig. 7 Electrochemical N 2 fixation. a Linear sweep voltammetric curves in N 2 -saturated (red line) and Ar-saturated (black line) electrolytes. b Yield of NH 3 production (red bars, left y axis) and Faradaic efficiency (green dots, right y axis) of Zr-TiO 2 at each given potentials. c 1 H nuclear magnetic resonance (NMR) analysis of the electrolyte fed by 15 N 2 (upper panel) and 14 N 2 (lower panel) after the electrolytic reactions. d Comparison of the ammonia yield rate (blue bars) and NH 3 Faradaic efficiencies (FE NH3 , green dots) using different feeding gases for the N 2 RR at − 0.45 V vs. RHE. e Yield of NH 3 (blue bars, left y axis) and FE NH3 (green dots, right y axis) of undoped TiO 2 at each given potentials. f Yields of NH 3 with different catalysts at − 0.45 V vs. RHE. (Source data are provided as a Source Data file.) Full size image The average yields of ammonia and the corresponding FE NH3 of those electrocatalysts were measured using the sodium salicylate-sodium hypochlorite method [13] (Methods section). The corresponding calibration plots were displayed (Supplementary Fig. 15 ). All samples were measured with over three times to get the average values. The quantification of ammonia was carefully controlled to avoid possible contamination sources [46] . To rule out the possible contamination of ammonia from the air or the solution, several control experiments were carried out, as specified in Supplementary Fig. 16 . Very little ammonia was detected in those controls, and the photographs of their colorimetric assays showed no color difference. In addition, as a control, the electrochemical tests were also conducted for all the electrocatalysts under Ar controls [47] . The corresponding ultraviolet-visible (UV–Vis) spectra of electrolyte after 3 h electrolysis and chromogenic reaction show the maximum values are comparable to the spectrum backgrounds (Supplementary Fig. 17 ), suggesting almost no ammonia was produced for all samples in an Ar-saturated electrolyte. For the electrochemical tests of Zr-TiO 2 conducted in N 2 -saturated electrolytes, the UV–Vis spectra show a significant enhancement of the peak centered around 660 nm, suggesting that the Zr-TiO 2 nanotubes catalyze N 2 reduction (Supplementary Fig. 18 ). No N 2 H 4 product is detected in the electrolyte for the Zr-TiO 2 catalysts after 3 h N 2 RR test (Supplementary Fig. 19 ). For the Zr-TiO 2 nanotubes, both the ammonia production rate and the corresponding FE NH3 reach their peak values at − 0.45 V vs. RHE, which are calculated as 8.90 ± 0.17 µg h −1 cm −2 catalyst and 17.3% (Fig. 7b ), respectively. Further increase the negative potential leads to the decrease of the ammonia production rate and FE NH3 , which can be attributed to the increase of the competitive HER on the electrode surfaces. The quantitative measurement of the ammonia production was further verified by two other methods, including the ion chromatography (IC) and the nuclear magnetic resonance (NMR) [48] . The 1 H NMR spectra show a triplet coupling (~ 52 Hz) for 14 NH 4 + and a doublet coupling (~ 72 Hz) for 15 NH 4 + (Fig. 7c ). The obtained ammonia production rate and the corresponding FE NH3 for 15 N 2 as the feeding gas are comparable to those used 14 N 2 (Fig. 7d and Supplementary Fig. 20 ), confirming that the ammonia detected is attributed to the electroreduction of N 2 . The total ammonia produced during the 3 h electrochemical reaction time was calculated as 0.538 μmol (detailed calculation shown in the Supplementary Note 2 ). In contrast, all the undoped TiO 2 (Fig. 7e ), Zr-rutile-TiO 2 (Supplementary Fig. 21 ), and Ce-TiO 2 (Supplementary Fig. 22 ) electrocatalysts exhibit much lower ammonia production rates, with the peak values of 1.48, 3.22, and 5.79 µg h −1 cm −2 catalyst at a higher negative potential of − 0.65 V, respectively. Furthermore, the N 2 RR tests were also conducted on ZrO 2 and CeO 2 nanoparticles under the same catalytic potential of − 0.45 V vs. RHE to probe the effect of Zr-incorporation (Fig. 7f ). Both the pure CeO 2 and ZrO 2 nanoparticles exhibit lower or even negligible NH 3 production rates. This comparison suggests that the bi-Ti 3+ pairs induced by Zr 4+ -doped TiO 2 function as excellent electrocatalytic centers for the N 2 fixation at ambient conditions. Finally, the chronoamperometry tests at selected applied potentials of − 0.5 and − 0.45 V (where the ammonia yields were the highest) show that the N 2 RR performance of the Zr-TiO 2 nanotubes catalyst was stable after several hours of continuous electrolysis (Supplementary Fig. 23 ). This cycling stability test was further repeated for a total of six runs (Supplementary Fig. 24 ), showing no obvious change in the NH 3 yield rate and current efficiency. After the electrochemical test, the Zr-TiO 2 catalyst was re-measured with XPS (Supplementary Fig. 25 ). No obvious difference is observed compared with that before the electrochemical test, further confirming the good stability of the Zr-TiO 2 nanotubes in N 2 RR electrocatalysis. In this work, we have first screened several types of Ti 3+ sites by means of DFT calculations. The adjacent bi-Ti 3+ pairs formed on the most-stable surface of anatase TiO 2 (i.e., A(101)-Vo) are identified as the active electrocatalytic centers, which can lead to a lying-down manner as efficient N 2 chemisorption and subsequent activation. However, similar bi-Ti 3+ pair sites formed on the most stable surface of rutile TiO 2 (i.e., R(110)-Vo), as well as the single Ti 3+ site, are concluded as the inactive sites. By further removing a second O 2‒ to form R(110)-2Vo, the adjacent bi-Ti 3+ pairs on rutile TiO 2 can now induce a lying-down chemisorption manner for N 2 (Supplementary Fig. 1b ), exhibiting a significant amount of negative charge on N 2 and an elongated N−N bond length. Nevertheless, as shown in Supplementary Fig. 1a and b, the formation of two adjacent Vo’s on rutile (110) surfaces is 0.36 eV higher than the formation of two separated Vo’s, downplaying the role of the adjacent bi-Ti 3+ sites on R(110)-2Vo. Hence the anatase (101) surface is the more suitable host for the development and enrichment of the active bi-Ti 3+ pair sites. 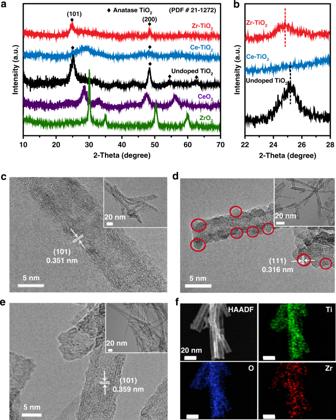Fig. 4 Structural and compositional characterizations.aX-ray diffraction (XRD) patterns of ZrO2, CeO2, undoped TiO2, Ce-TiO2, and Zr-TiO2.bThe enlarged view of XRD pattern at 22o−28orange.c–eHigh-resolution transmission electron microscopy (HRTEM) images ofcundoped TiO2,dCe-TiO2, andeZr-TiO2samples. Insets: Transmission electron microscopy (TEM) images of the corresponding nanotubes.fHigh-angle annular dark-field scanning transmission electron microscopy (HAADF-STEM) image with corresponding element mappings of Zr-TiO2, showing the distribution of Ti (green), O (blue), and Zr (red). (Source data are provided as a Source Data file.) The competitive adsorption of H 2 O and activation of HER on these bi-Ti 3+ catalytic sites are also estimated (Supplementary Table 4 ). For convenience, here we assume the chemical potential of the water in solution is equal to 3.169 kPa as pure liquid water at room temperature. Then, the calculated adsorption free energy changes is only 0.04 eV, when the adsorbed H 2 O on the bi-Ti 3+ sites is replaced by the N 2 under working condition (the corresponding structures are presented in Supplementary Fig. 26 ). For HER, the adsorption free energy of the first hydrogen is calculated to be 0.19 eV on the oxygen vacancy, which is only slightly more advantageous than that of N 2 RR of 0.24 eV. Meanwhile, one has to take into account the fact that the high pH of the electrolyte (pH 13) has an inhibiting effect on the HER [46] . Thus, N 2 in our situation is able to compete with H 2 O and H for adsorption and activation as shown in our experiments. In addition, previous literatures show that if the anatase nanoparticles are exposed under reduction situation with hydrogen, it results in reduced nanoparticles comprising a crystalline TiO 2 core and a disordered shell with abundant oxygen vacancies [49] . With respect to the corresponding pristine surface O*, the calculated free energy diagrams for the further reduced surface OH* and H 2 O* of pristine A(101) surface, with and without Zr-doping under different potentials, are shown in Supplementary Fig. 27 . The result suggests that the surface with O* totally hydrogenated is the most stable under working conditions for U RHE < −0.40 eV, such that the oxygen vacancies should remain thermodynamically stable, which should not be annihilated by the O** or OH* species. As Zr 4+ is not a reducible cation, it is not expected to directly form Vo’s next to Zr 4+ , but our work shows that the doping of Zr 4+ into the anatase TiO 2 framework is a useful strategy to induce and enrich the specific adjacent bi-Ti 3+ pairs on the anatase surfaces. Owing to its similar d -electron configuration and oxide structure but relatively larger ionic size as compared with Ti 4+ , the doped single Zr 4+ ion induces a strained effect without breaking the original TiO 2 structure, which, in turn, enhances the formation of oxygen vacancy and subsequently bi-Ti 3+ sites on the anatase surfaces. Control experiments reveal that Ce 4+ doping does not have the same role as Zr 4+ doping, for Ce 4+ has a too larger size and a variable oxidation state. Based on an expanded anatase lattice with lattice constants that are 1.023 times larger than the optimized one by DFT, various anatase A(101) surfaces were built without or with different Zr 4+ concentrations in surfaces or subsurfaces. The calculated results for some representatives of the strained A(101) surfaces are shown in Supplementary Table 3 . The Vo formation energy without Zr 4+ doping is calculated to be 0.27 eV lower than the A(101) surface based on the optimized lattice. With various contents of Zr 4+ dopants in surfaces or subsurfaces, the calculated Vo formation energies are within 0.22 and 0.33 eV smaller than that of the optimized lattice. The DFT results support the experiment observation that Zr 4+ enhances the Vo formation on A(101) surface, which is owing to the tensile strain induced by the Zr 4+ doping. Owing to the efficient chemisorption and activation of the N 2 molecules by the Zr 4+ doping-induced bi-Ti 3+ pairs on anatase TiO 2 , the Zr-TiO 2 exhibits an outstanding ammonia production rate, a high FE NH3 , and excellent electrochemical stability, significantly exceeding those of the undoped TiO 2 or Ce-TiO 2 samples under similar testing conditions. 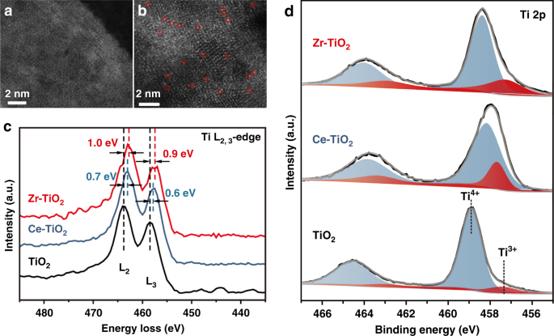Fig. 5 Structural and compositional characterizations. High-angle annular dark-field scanning transmission electron microscopy (HAADF-STEM) ofaundoped TiO2andbZr-TiO2samples. Single Zr4+ions were highlighted by red circles.cElectron energy loss spectroscopy (EELS) profiles of the Ti-L2, 3edge recorded across the undoped TiO2, Ce-TiO2, and Zr-TiO2samples.dTi 2p X-ray photoelectron spectroscopy (XPS) spectra of the Zr-TiO2, Ce-TiO2, and undoped TiO2, samples. (Source data are provided as a Source Data file.) Compared with other N 2 RR electrocatalysts in aqueous solutions at ambient conditions reported to date (Supplementary Table 5 ), our Zr-TiO 2 sample demonstrated one of the highest NH 3 production rates and FE NH3 values. In conclusion, our study demonstrates the bonding nature of the active centers and a unique approach of optimizing electrocatalytically active sites by rational design of dopant size and charge, enabling new opportunities for efficient electrochemical N 2 reduction. Our work not only reveals bi-Ti 3+ pairs on anatase TiO 2 as effective N 2 RR active centers, but also suggests an attractive viewpoint to understand and apply the same-valance dopants in heterogeneous catalysis, which is generally useful but still poorly understood. Further development of similar multiple active sites with cooperative binding and activation effects on N 2 may lead to a vast variety of opportunities of enhancing the N 2 RR capabilities and potential large-scale utilization toward direct atmospheric N 2 fixation. Chemicals and materials Titanium (IV) oxide (P25, Sinopharm Chemical Reagent Co., Ltd, analytically pure), zirconium nitrate pentahydrate (Aladdin, Z190748, 99.5%), cerium nitrate hexahydrate (Aladdin, C105378, 99.5%), sodium hydroxide (Macklin, S817977, ≥ 98%), salicylic acid (Macklin, S817529, 99.5%), potassium sodium tartrate tetrahydrate (Macklin, P816438, 99.5%), sodium nitroferricyanide(III) dehydrate (Macklin, S818341, 99.98% metals basis), sodium hypochlorite solution (Macklin, S828471, available chlorine 4.0%), ammonium chloride (Maclin, A801305, 99.8%), hydrazine monohydrate (Alfa Aesar, A14005, 98%), hydrochloric acid (Sinopharm Chemical Reagent Co., Ltd, 10011018, 36.0−38.0%), potassium hydroxid (Aladdin, P112287, 99.99% metals basis), sulfuric acid (Sinopharm Chemical Reagent Co., Ltd, 10021618, 95.0−98.0%), ethyl alcohol (Sinopharm Chemical Reagent Co., Ltd, 10009218, ≥ 99.7%), 4-(dimethylamino) benzaldehyde (Sigma-Aldrich, 156477, 99%), Nafion solution (Dupont), 211 Nafion membrane (Dupont), deionized (DI) water (Millipore, 18.2 MΩ cm), N 2 gas (99.99%), Ar gas (99.99%). Ammonium sulfate ((NH 4 ) 2 SO 4 , 99%), ( 15 NH 4 ) 2 SO 4 , 98 atom% 15 N), and nitrogen- 15 N 2 (98 atom% 15 N) were purchased from Sigma-Aldrich. All chemical reagents were used as received without further purification. Characterization The XRD data were characterized by Bruker SMART APEX (II)-CCD (Germany). X-ray photoelectron spectroscopy was recorded on a Perkin Elmer PHI 5000 C ESCA system (Perkin Elmer, USA). The high-resolution transmission electron microscopy images and the EDX spectroscopy spectra were recorded by a JEM 2100 F (JEOL, Japan) and a Tecnai T20 (FEI, USA) transmission electron microscope. The HAADF-STEM, EELS, and the EDX mapping experiments were performed using Titan Cubed Themis G2 300 (FEI) microscope equipped with Super-X detectors at 200 kV. N 2 -TPD measurements were performed on a Micrometrics Autochem II 2920 system. Electron-spin resonance signals were recorded on a Bruker ESR A300 spectrometer at room temperature. XANES and EXAFS data were collected on beamline 14 W at the Shanghai Synchrotron Radiation Facility (SSRF). The UV–Vis absorption spectrum was recorded by an ultraviolet-visible spectrometer (U-3900H, Hitachi, Japan). 1 H-NMR (nuclear magnetic resonance) measurements were performed on a Bruker NMR600. IC analysis was performed on an ICS-2000 (Thermo Fisher Scientific) equipped with an isocratic pump. Synthesis of Zr-TiO 2 In a typical synthesis, 2.0 g of TiO 2 (P25) was mixed with 60 mL of (10 m ) NaOH solution in a Teflon-lined stainless autoclave at 150 °C for 20 h. The slurry was washed with 0.1 m HCl solution for several times until the pH value reached 1.6, and then with DI water until pH was close to 7, before being filtrated to obtain TiO 2 nanotubes. The introduction of Zr 4+ to TiO 2 was conducted by wet impregnating the TiO 2 nanotubes with 20 mL of 0.35 m zirconium nitrate solution. The mixture was stirred at room temperature for 4 h. After the reaction, the substrate was washed with DI water and ethanol for several times, followed by drying at 60 °C and then annealed in Ar at 400 °C, with a ramping rate of 2 °C min ‒1 for 2.5 h. Electrochemical measurements A total of 5 mg of catalyst was dispersed in 0.5 mL of ethanol followed by the addition of 50 µL of Nafion solution. The mixture was sonicated thoroughly to form a homogeneous ink. The working electrodes were then prepared by drop-casting the catalyst inks onto carbon paper to achieve a loading of 1.0 mg cm ‒2 . All the electrochemical performance measurements were performed with an Autolab electrochemical workstation (Autolab PGSTAT204) at room temperature (25 ± 2 °C) using 0.1 m KOH as the electrolyte. For the electrocatalytic N 2 RR, a saturated calomel electrode (SCE) and a Pt wire were used as reference and counter electrodes, respectively. The potentials were all converted to the RHE scale according to Nernst equation ( 1 ): 
    E_RHE( V) = E_SCE( V) + E^o_SCE( V) + 0.0591 ×pH = E_SCE( V) + 1.008 V
 (1) where E RHE is the converted potential vs. RHE, E SCE is the experimental potential measured vs. SCE, E 0 SCE is the standard potential of SCE at 25 °C. The potential of SCE was calibrated to the RHE in 0.1 m KOH electrolyte saturated with high-purity H 2 (Supplementary Fig. 11 ), consistent with the Equation ( 1 ). The scan rate for LSV was kept at 1.0 mV s ‒1 . For the potentiostatic measurement, the KOH electrolyte (pH 13, 30 mL) was purged with pure N 2 for 30 min before the measurement. For comparison, the same electrochemical test was also conducted in an Ar-saturated KOH solution. Constant potential electrolysis was conducted at various potentials for 3 h. The electrochemical experiments were repeated for three times to obtain the averaged measured values. Determination of ammonia The concentration of produced ammonia was spectroscopically determined by the indophenol blue method [50] with some modification. Sodium salicylate (5 g), sodium hydroxide (1.47 g), and potassium sodium tartrate tetrahydrate (5 g) were dissolved in DI water and diluted to 100 mL was used as the color reagent A. In brief, 8 mL of the testing electrolyte was taken from the electrochemical cell, followed by adding 1 mL of color reagent A, 100 μL of (10 mg/mL) sodium nitroferricyanide (C 5 FeN 6 Na 2 O), and 100 μL of 0.05 m NaClO. The UV-Vis absorption spectra were then measured. The concentration of indophenol blue was determined using the absorbance at 660 nm. The concentration-dependence absorption curves were calibrated using standard ammonia chloride solutions with different concentrations. All the spectroscopic measurements were repeated for three times to obtain the averaged measured values. The fitting curve ( y = 0.1066 x + 0.0109, R 2 = 0.9991) showed good linear relation of absorbance value with NH 3 concentrations. Determination of NH 3 yield rate and FE NH3 The electrochemical ammonia yield rate ( r NH3 (electrochemical) ) was calculated by subtracting the background signal of non-electrochemical ammonia, using Equation ( 2 ): 
    r_NH3 ( electrochemical) = Δ c_NH_3 (yield)× V_aq/t × A
 (2) where Δ c NH3 (yield) = c NH3 (yield, N2) − c NH3 (yield, Ar) . c NH3 (yield, N2) is the measured NH 4 + mass concentration in an N 2 -saturated electrolyte, c NH3 (yield, Ar) is the measured NH 4 + mass concentration in an Ar-saturated electrolyte as a control. V aq is the volume of electrolyte, t is the electrochemical reaction time, and A is the geometric area of the cathode. The electrochemical ammonia faradaic efficiency ( FE NH3 (electrochemical) ) was calculated by subtracting the background signal of non-electrochemical ammonia [47] , using Equation ( 3 ): 
    FE_NH3 ( electrochemical) = n ×Δ c_NH__3 (yield)× V_aq× F/17× Q×100 %
 (3) where n is the number of transferred electrons (3), F is the Faraday constant, and Q is the quantity of applied electric charges. In order to identify the source of ammonia, 15 N 2 enriched gas was employed to serve as the feeding gas. After N 2 reduction reaction, the NH 4 + -containing electrolyte was characterized by 1 H NMR measurement, using 1 m m maleic acid as an internal standard. 10% dimethyl sulphoxide (DMSO)- d 6 was used as the solvent. A doublet coupling (~ 72 Hz) for 15 NH 4 + and a triplet coupling (~ 52 Hz) for 14 NH 4 + were observed for different testing solutions. For the IC method, 3 mL of electrolyte was transferred into the chromatograph. The sample loop was 20 μL, with methanesulfonic acid as the eluent. The concentration-dependence plot by the IC method was characterized with different standard NH 4 + concentrations. Note that specific precautions were necessary with rigorous control experiments to minimize possible ammonia contamination during the N 2 RR test [46] . (1) The chemicals including water were purchased or prepared with high purity. (2) All the electrochemical measurements including control experiments were conducted at fume hoods to provide a clean atmosphere. (3) Considering the effect of human respiration and skin contaminates, masks and latex gloves (pre-soaked in 100 mL of 0.01 m HCl for 3 h) were used during the N 2 RR tests and ammonia quantification measurement. Determination of hydrazine The hydrazine presented in the electrolyte was estimated by the method of Watt and Chrisp [51] . A mixture of para-(dimethylamino) benzaldehyde (5.99 g), HCl (concentrated, 30 mL) and ethanol (300 mL) was used as a color reagent B. In brief, 5 mL of testing electrolyte after the electrocatalytic reaction was taken out from the electrochemical cell, followed by adding 5 mL of color reagent B. 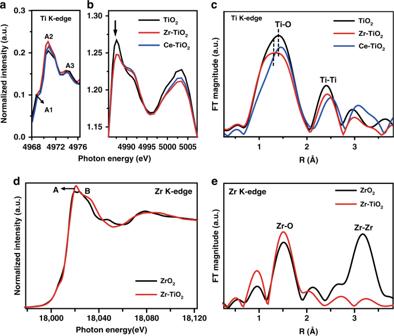Fig. 6 X-ray absorption spectroscopy characterizations.a,bEnlarged TiK-edge X-ray absorption near-edge structure (XANES) spectra, andcFourier transformed (FT)k3-weighted of TiK-edge Extended X-ray Absorption Fine Structure (EXAFS) spectra of the undoped TiO2, Zr-TiO2, and Ce-TiO2samples.dZrK-edge XANES spectra andeFourier-transformedk3-weighted of EXAFS spectra of pure ZrO2and Zr-TiO2samples. (Source data are provided as a Source Data file.) 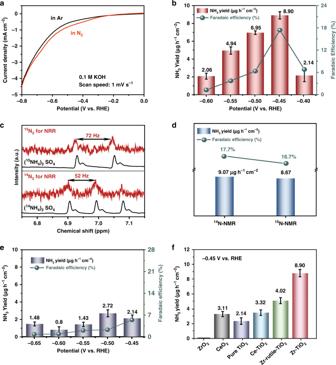Fig. 7 Electrochemical N2fixation.aLinear sweep voltammetric curves in N2-saturated (red line) and Ar-saturated (black line) electrolytes.bYield of NH3production (red bars, leftyaxis) and Faradaic efficiency (green dots, rightyaxis) of Zr-TiO2at each given potentials.c1H nuclear magnetic resonance (NMR) analysis of the electrolyte fed by15N2(upper panel) and14N2(lower panel) after the electrolytic reactions.dComparison of the ammonia yield rate (blue bars) and NH3Faradaic efficiencies (FENH3, green dots) using different feeding gases for the N2RR at − 0.45 V vs. RHE.eYield of NH3(blue bars, leftyaxis) and FENH3(green dots, rightyaxis) of undoped TiO2at each given potentials.fYields of NH3with different catalysts at − 0.45 V vs. RHE. (Source data are provided as a Source Data file.) After 20 min for color development, the UV-Vis absorption spectra were measured at 455 nm. The concentration-dependence plot was obtained by using standard hydrazine monohydrate solutions with different concentrations. The fitting curve showed good linear relation of absorbance with N 2 H 4 ·H 2 O concentration ( y = 0.7624 x + 0.0161, R 2 = 0.9992) by three times independent calibrations. Computational details The Vienna ab initio simulation package was utilized to perform all DFT calculations [52] , [53] , [54] . The 2 s , 2 p electrons in oxygen and nitrogen, the 3 d , 4 s electrons in titanium and the 5 s , 4 d , 5 p electrons in zirconium were treated as valence electrons, whereas the kinetic energy cutoff for the plane wave basis sets was set to be 400 eV. The remaining core electrons were described by the projector augmented-wave method [55] . The surface Monkhorst–Pack meshes [56] of 2 × 2 × 1 and 5 × 5 × 5 k -point sampling in the surface Brillouin zone were employed for slab model and bulk, respectively. For bulk optimization, all atoms as well as lattice constants were allowed to fully relax. For systems involving anatase (101), a 1 × 3 supercell of 12 atomic layers was used, where the bottom five layers of atoms were fixed in their optimized bulk positions, whereas the top seven layers, as well as the adsorbate, were allowed to fully relax. For systems involving rutile (110), a 3 × 2 supercell of 12 atomic layers was used, where the bottom five layers of atoms were fixed in their optimized bulk positions, whereas the top seven layers, as well as the adsorbate, were allowed to fully relax. After the convergence criteria for optimizations were met, the largest remaining force on each atom was less than 0.02 eV Å ‒1 . For all calculations, the spin polarized generalized gradient approximation of the Perdew–Burke–Ernzerhof functional [57] was used. As the standard DFT functions tended to over-delocalize electrons, DFT + U was employed [58] with an effective U value of 3.3 eV for Ti 3 d -orbitals, as obtained from linear response [59] . For the dopants, we used standard DFT on Zr, as there were no issues with describing the electronic structure [21] . For surface reactions, the contributions of dispersive interactions were accounted for by using the DFT + D3 method with Becke-Jonson damping [60] , [61] . Bader’s theory of atoms in molecules was used for charge analysis [30] , [62] , [63] . Oxygen vacancy formation energies were calculated as: 
    Δ E( Vo) = E_t( Ti_xO_2x-1) + 1/2 E_t( O_2)-E_t( Ti_xO_2x)
 (4) where E t (Ti x O 2x-1 ) and E t (Ti x O 2x ) are the total energies of the optimized supercell with and without V O vacancy, respectively, and E t (O 2 ) is the total energy of a gas phase O 2 . The second Vo formation energies, from Ti x O 2x-1 were calculated as: 
    Δ E( Vo) = E_t( Ti_xO_2x-2) + 1/2 E_t( O_2)-E_t( Ti_xO_2x-1)
 (5) where E t (Ti x O 2x-2 ) is the total energies of the optimized supercell with the first and second V O vacancy, respectively. This type of oxygen vacancy formation energy is commonly used in theoretical heterogeneous catalysis, as it is convenient to compare different oxides (doped or undoped) under different reaction conditions [18] . Indeed, the formation of oxygen vacancies in reducible oxides like TiO 2 and CeO 2 is relatively easy [18] , in particular, under the reduction conditions such as H 2 or CO atmosphere, or on the anode surfaces as in the present work. The formation energy of oxygen vacancies should be related with H 2 O or CO 2 formation, thus providing the thermodynamic driving force. The adsorption free energies of gases on the surfaces were calculated as: 
    Δ G( gas) = G_t( gas/surface)-G_t( gas)-G_t( surface),
 (6) where G t (gas/surface), G t (surface), and G t (gas) are the total free energies of the adsorption systems of surfaces with or without vacancies, and adsorbate species in the gas phase, respectively. Here, we assumed that in addition to the total electronic energies, only the translation and rotation contributions of the gas phase species are significant and the other parts can be ignored. Assuming the gas phase species as ideal gases, the partition functions of translation Q trans and rotation Q rot were calculated as: [64] 
    Q_A^trans = ( 2πm_Ak_BT/h^2)^3/2V
 (7) 
    Q_A^rot = 1/σ( k_BT/h)^3/2√(π/A^rotB^rotC^rot)
 (8) where P (1 atm) and m are the partial pressure and molecular mass, respectively, k B is the Boltzmann constant, T (298.15 K) is the absolute temperature, \(V = \frac{{k_{\mathrm{B}}T}}{{P_{\mathrm{A}}}}\) is the volume of the system, σ is the symmetry factor, A rot , B rot , C rot are rotational constants, and h is the Plank’s constant. In our work, the DFT calculations were carried out to rationally screen four types of Ti 3+ for a better understanding of bonding structures of the active centers (Fig. 2 ): (a) the adjacent bi-Ti 3+ on anatase (101) surfaces with one oxygen vacancy (i.e., A(101)-Vo); (b) the single Ti 3+ with four coordination on anatase (101) surfaces with one oxygen vacancy; (c) the adjacent bi-Ti 3+ on rutile (110) surfaces with one oxygen vacancy, (i.e, R(110)-Vo); (d) the adjacent bi-Ti 3+ on rutile (110) surfaces with a pair of oxygen vacancies together, (i.e., R(110)-2Vo’s). Cases (a) and (c) were chosen because anatase and rutile are the most common crystal phases for TiO 2 , and anatase (101) and rutile (110) surfaces are, respectively, the most exposed surfaces. Case (b) was chosen for its low coordination. Case (d) was formed after the removal of one nearby lattice O 2‒ in Case (c). This nearby lattice O 2‒ presents a large repulsion with the chemisorbed N 2 in a lying-down manner, which precludes the bi-Ti 3+ site of R(110)-Vo from effective N 2 activation. The overall N 2 RR process (N 2 + 6 H + + 6e ‒ → 2NH 3 ) involves several proton-coupled electron transfer steps. The Gibbs free energy change (Δ G ) of each elementary step was calculated by using the standard hydrogen electrode model [27] , [28] , [65] , which uses one-half of the chemical potential of hydrogen as the chemical potential of the proton-electron pair. According to this method, the Δ G value can be determined as: 
    Δ G = Δ H-TΔ S + Δ G_U + Δ G_pH
 (9) where Δ H and Δ S are the enthalpy change and entropy change, respectively. Δ G U is the free energy contribution related to electrode potential U. Δ G pH is the correction of the H + free energy by the concentration, which can be calculated as 
    Δ G_pH = 2.303 × k_BT×pH
 (10)